Hepatic insulin signalling is dispensable for suppression of glucose output by insulinin vivo Insulin signalling and nutrient levels coordinate the metabolic response to feeding in the liver. Insulin signals in hepatocytes to activate Akt, which inhibits Foxo1 suppressing hepatic glucose production (HGP) and allowing the transition to the postprandial state. Here we provide genetic evidence that insulin regulates HGP by both direct and indirect hepatic mechanisms. Liver-specific ablation of the IR ( L -Insulin Receptor KO) induces glucose intolerance, insulin resistance and prevents the appropriate transcriptional response to feeding. Liver-specific deletion of Foxo1 (L-IRFoxo1DKO) rescues glucose tolerance and allows for normal suppression of HGP and gluconeogenic gene expression in response to insulin, despite lack of autonomous liver insulin signalling. These data indicate that in the absence of Foxo1, insulin signals via an intermediary extrahepatic tissue to regulate liver glucose production. Importantly, a hepatic mechanism distinct from the IR–Akt–Foxo1 axis exists to regulate glucose production. The dynamic regulation of liver glucose metabolism is essential for systemic carbohydrate homeostasis and organismal survival. During times of starvation, the liver produces the amount of glucose necessary to meet the metabolic demands of the body. This increased hepatic glucose production (HGP) during fasting results from an initial breakdown of glycogen stores before transitioning to gluconeogenesis from various precursors. In the postprandial state, this process is opposed by the rise of the hormone insulin, which suppresses HGP. However, in insulin-resistant disorders such as diabetes, insulin fails to regulate HGP, leading to elevated circulating glucose concentrations [1] , [2] . Various models have been proposed to explain the inability of insulin to suppress HGP during diabetes, though there is still no consensus for the mechanism. Prevalent hypotheses include increased delivery of gluconeogenic precursors and fatty acids to the liver, accumulation of neutral lipids in liver, altered systemic cytoadipokines, distorted glucagon-to-insulin ratios, and defective hepatic insulin signalling [3] . Since excess HGP drives fasting hyperglycaemia in diabetes, the elucidation of the mechanisms of how insulin regulates hepatic metabolism in normal and pathological livers has received substantial attention. In liver, insulin signals through its receptor (IR), insulin receptor substrates (Irs) and phosphoinositide 3′-kinase to activate the serine/threonine kinase Akt, which utilizes several distinct downstream pathways to modulate liver metabolism [4] . In hepatocytes, insulin promotes protein translation and cell growth by activating the mammalian target of rapamycin complex 1 (mTORC1) via Akt-mediated phosphorylation and inactivation of the tuberous sclerosis protein 1 and 2 complex [5] . Insulin also induces lipogenesis and glycogen synthesis via Akt-dependent mechanisms [6] , [7] , [8] . Finally, insulin stimulates an Akt-dependent inhibitory phosphorylation of Foxo1, which is thought to be the master regulator of key gluconeogenic genes leading to the subsequent regulation of glucose output [9] , [10] , [11] , [12] , [13] , [14] . In support of this notion, ablating hepatic Foxo1 in insulin-resistant models improves glucose homeostasis [15] , [16] . However, deletion of liver Foxo1 in lean mice only modestly reduces fasting glucose and hypoglycemia occurs only after prolonged fasting, leading to uncertainty concerning the role of Foxo1 in normal liver glucose metabolism [11] , [17] . A reduction of the IR–IRS–Akt pathway activity in mouse livers results in glucose intolerance, systemic insulin resistance and a failure to suppress appropriately glucose production in response to insulin [15] , [17] , [18] . Concomitant deletion of Foxo1 normalizes the glucose intolerance and hyperinsulinemia triggered by hepatic deletion of Irs or Akt [15] , [17] . Surprisingly, mice with liver-specific deletion of Akt and Foxo1 (L-AktFoxo1TKO) still respond to insulin in vivo by suppressing gluconeogenic gene expression and HGP. Furthermore, L-AktFoxo1TKO mice adapt appropriately to the postprandial state despite lacking canonical liver insulin signalling [17] . These data are inconsistent with the established model of hepatic insulin action and suggest Akt is not an obligate intermediate for insulin action under all conditions. Importantly, these data suggest the existence in liver of a signalling pathway parallel to the Akt–Foxo1 axis that is capable of regulating HGP. At least two alternative mechanisms can be formulated to explain the insulin effects in L-AktFoxo1TKO mice: (1) insulin acts directly on the liver via the IR–Irs pathway; however, a bifurcation occurs before Akt thereby activating an unidentified parallel pathway independent of Akt to suppress HGP [19] ; or (2) insulin acts non-autonomously via a peripheral tissue to regulate HGP. In the study reported in this manuscript, we tested the second hypothesis by deleting insulin receptor specifically and exclusively in liver, with and without concomitant deletion of Foxo1 . We reasoned that if insulin were suppressing HGP by acting via an intermediary, non-hepatic cell type, which then sends a signal to liver, the effect of insulin should not depend on the presence of its receptor on hepatocytes. Acute liver-specific deletion of IR To minimize potential secondary and/or compensatory responses from congenital hepatic insulin receptor (IR) deficiency, we generated a model of acute, liver-specific knockout of the IR . Adult IR loxP/loxP mice were injected with an adeno-associated virus containing a liver-specific promoter (thyroxine-binding globulin) driving Cre recombinase to delete the IR (L-Insulin Receptor KO) [8] . IR loxP/loxP (LWT) mice injected with virus expressing GFP instead of Cre served as a control. A western blot confirmed efficient deletion of IR in primary hepatocytes isolated from mice following the virus injection ( Fig. 1a ). Akt phosphorylation at Ser473 in response to insulin was undetectable in hepatocytes isolated from L-Insulin Receptor KO mice. In contrast to the major metabolic abnormalities reported in the congenital IR liver knockout mouse (LIRKO) [18] , L-Insulin Receptor KO mice displayed normal fasting glucose levels ( Fig. 1b ) and modest postprandial hyperglycaemia following 4 h of refeeding ( Fig. 1c ). As expected, L-Insulin Receptor KO mice were glucose intolerant ( Fig. 1d ) and hyperinsulinemic following fasting and 15 min following an intraperitoneal glucose injection ( Fig. 1e ). 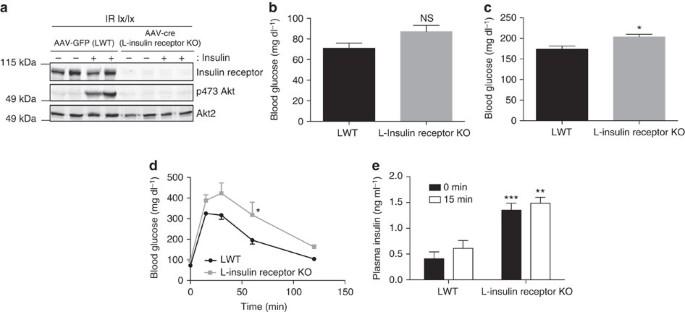Figure 1: Acute deletion of liver insulin receptor leads to glucose intolerance and insulin resistance. (a) Western blot of primary hepatocytes from mice treated with 10 nM insulin for 15 min and probed for specific proteins as indicated. AAV-GFP=LWT mice, AAV-Cre=L–Insulin Receptor KO mice. (b,c) Blood glucose concentrations in mice after overnight fast (b) and overnight fasted following by 4 h refeeding of normal chow (c). NS, not significant *P<0.05.n=5 mice. (d) Intraperitoneal glucose tolerance test (2 g kg−1) on overnight fasted mice.n=5 mice per group. *P<0.05 versus LWT. Statistical analysis was performed two-way analysis of variance followed by Bonferroni when two conditions were involved. (e) Insulin levels before and after 15 min following glucose injection IP.n=5 mice per group. ***P<0.001, **P<0.01 versus LWT. All the data are presented as mean±s.e.m. Statistical analysis was performed using Students’st-test followed by two-tailed analysis. AP<0.05 was considered statistically significant. Figure 1: Acute deletion of liver insulin receptor leads to glucose intolerance and insulin resistance. ( a ) Western blot of primary hepatocytes from mice treated with 10 nM insulin for 15 min and probed for specific proteins as indicated. AAV-GFP=LWT mice, AAV-Cre=L–Insulin Receptor KO mice. ( b , c ) Blood glucose concentrations in mice after overnight fast ( b ) and overnight fasted following by 4 h refeeding of normal chow ( c ). NS, not significant * P <0.05. n =5 mice. ( d ) Intraperitoneal glucose tolerance test (2 g kg −1 ) on overnight fasted mice. n =5 mice per group. * P <0.05 versus LWT. Statistical analysis was performed two-way analysis of variance followed by Bonferroni when two conditions were involved. ( e ) Insulin levels before and after 15 min following glucose injection IP. n =5 mice per group. *** P <0.001, ** P <0.01 versus LWT. All the data are presented as mean±s.e.m. Statistical analysis was performed using Students’s t -test followed by two-tailed analysis. A P <0.05 was considered statistically significant. Full size image Hepatic Foxo1 deletion in L-Insulin Receptor KO mice Insulin signals via its receptor to activate Akt and suppress Foxo1-dependent transcription. Hepatic Foxo1 deletion reverses the metabolic abnormalities resulting from liver-specific knockout of Irs or Akt [15] , [17] . To determine whether constitutive Foxo1 activation is responsible for the abnormal glucose metabolism following hepatic IR deletion, adult IR loxP/loxP ;FoxO1 loxP/loxP mice were injected with AAV-Tbg-Cre to generate liver-specific deletion of IR and Foxo1 (L-IRFoxo1DKO). Mice injected with virus expressing GFP instead of Cre served as controls (LWT). A western blot confirmed excision of the IR and Foxo1 in primary hepatocytes and liver lysates from L-IRFoxo1DKO mice ( Fig. 2a ). L-Insulin Receptor KO and L-IRFoxo1DKO mice failed to activate canonical insulin targets (phosphorylation of Akt, S6 and PRAS40) following a supraphysiological dose of insulin ( Fig. 2b ). However, feeding elicited significant S6 phosphorylation in all genotypes, supporting the notion that hepatic IR is not required for the activation of the mTorc1 complex by nutrients ( Fig. 2c ) [20] . Concomitant deletion of Foxo1 restored Igfbp1 protein to LWT levels, while also partially increasing glucokinase protein concentration albeit not to the levels present in LWT mice ( Fig. 2c ). Deletion of Foxo1 normalized the fasting ( Fig. 2d ) and postprandial hyperglycaemia in the L-Insulin Receptor KO ( Fig. 2e ). In addition, L-IRFoxo1DKO mice demonstrated improved glucose tolerance ( Fig. 2f ) and Foxo1 deletion rescued the hyperinsulinemia caused by hepatic deletion of the IR ( Fig. 2g ). The relatively normal metabolic phenotype of the L-IRFoxo1DKO mice was assessed in an alternative model, that is, the congenital liver-specific knockout generated with a liver-specific Cre transgene. Consistent with data with acute recombination, deletion of Foxo1 normalized the glucose intolerance caused by liver-specific deletion of IR ( Fig. 2h ). These data support the concept that a significant increase in Foxo1 activity in the L-Insulin Receptor KO mice as a result of defective Akt activation is responsible for the diabetic-like phenotype of the L-Insulin Receptor KO mice. 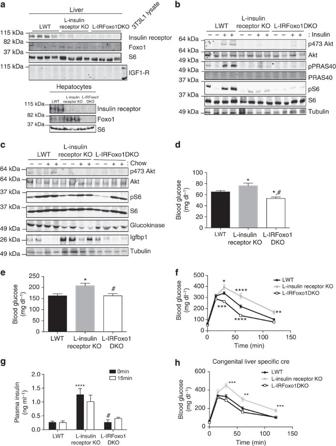Figure 2: LiverFoxo1deletion normalizes glucose levels and hyperinsulinemia in L-Insulin Receptor KO mice despite lack of hepatic insulin signalling. (a) Western blot from primary hepatocyte and liver lysates of mice from indicated gentoypes probed for specific proteins as indicated. (b) Western blot of liver lysates in mice fasted overnight and i.p. injected with either saline or insulin (2 mU g−1) and probed for specific proteins as indicated. (c) Western blot of liver lysates in mice fasted overnight and refed normal chow for 4 h and probed for specific proteins as indicated. (d,e) Blood glucose concentrations in mice after overnight fast (d) and overnight fasted following by 4 h refeeding of normal chow (e). *P<0.05 versus LWT, #P<0.0001 versus L-Insulin Receptor KO. LWT group includes total of 18 mice in fasting group withn=10IRloxP/loxPandn=8IRloxP/loxP;Foxo1loxP/loxPand in refed group includes total of 9 mice in fasting group withn=4IRloxP/loxPandn=5IRloxP/loxP;Foxo1loxP/loxP. L-Insulin Receptor KO includesn=12 for fasting group andn=6 for refed group. L-IRFoxo1DKO includesn=22 for fasting group andn=7 for refed group. (f) Intraperitoneal glucose tolerance test (2 g kg−1) on overnight fasted mice. LWT group includes total of eight mice withn=6IRloxP/loxPandn=2IRloxP/loxP;Foxo1loxP/loxP. L-Insulin Receptor KO includesn=7 and L-IRFoxo1DKO includesn=8. *P<0.05 versus LWT, ****P<0.0001 versus LWT (g) Insulin levels before and after 15 min following glucose injection. LWT group includes total of eight mice withn=6IRloxP/loxPandn=2IRloxP/loxP;Foxo1loxP/loxP, L-Insulin Receptor KO includesn=6 and L-IRFoxo1DKO includesn=13, for fasting group. LWT group includes total of three mice withn=2IRloxP/loxPandn=1IRloxP/loxP;Foxo1loxP/loxP, L-Insulin Receptor KO includesn=3 and L-IRFoxo1DKO includesn=8 for 15 min group. ****P<0.0001 versus LWT, # toP<0.0001 vs L-Insulin Receptor KO (h) Intraperitoneal glucose tolerance test (2 g kg−1) on overnight fasted mice.n=7–10 mice. LWT group includes total of six mice withn=5IRloxP/loxPandn=1IRloxP/loxP;Foxo1loxP/loxP. L-Insulin Receptor KO includesn=8 and L-IRFoxo1DKO includesn=5. **P<0.01 versus LWT, ****P<0.0001 versus LWT. All data are presented as mean±s.e.m. Statistical analysis was performed using one-way analysis of variance followed by Tukey post-test when more than two groups were compared, two-way analysis of variance followed by Bonferroni when two conditions were involved. AP<0.05 was considered statistically significant. Figure 2: Liver Foxo1 deletion normalizes glucose levels and hyperinsulinemia in L-Insulin Receptor KO mice despite lack of hepatic insulin signalling. ( a ) Western blot from primary hepatocyte and liver lysates of mice from indicated gentoypes probed for specific proteins as indicated. ( b ) Western blot of liver lysates in mice fasted overnight and i.p. injected with either saline or insulin (2 mU g −1 ) and probed for specific proteins as indicated. ( c ) Western blot of liver lysates in mice fasted overnight and refed normal chow for 4 h and probed for specific proteins as indicated. ( d , e ) Blood glucose concentrations in mice after overnight fast ( d ) and overnight fasted following by 4 h refeeding of normal chow ( e ). * P <0.05 versus LWT, # P <0.0001 versus L-Insulin Receptor KO. LWT group includes total of 18 mice in fasting group with n =10 IR loxP/loxP and n =8 IR loxP/loxP ;Foxo1 loxP/loxP and in refed group includes total of 9 mice in fasting group with n =4 IR loxP/loxP and n =5 IR loxP/loxP ;Foxo1 loxP/loxP . L-Insulin Receptor KO includes n =12 for fasting group and n =6 for refed group. L-IRFoxo1DKO includes n =22 for fasting group and n =7 for refed group. ( f ) Intraperitoneal glucose tolerance test (2 g kg −1 ) on overnight fasted mice. LWT group includes total of eight mice with n =6 IR loxP/loxP and n =2 IR loxP/loxP ;Foxo1 loxP/loxP . L-Insulin Receptor KO includes n =7 and L-IRFoxo1DKO includes n =8. * P <0.05 versus LWT, **** P <0.0001 versus LWT ( g ) Insulin levels before and after 15 min following glucose injection. LWT group includes total of eight mice with n =6 IR loxP/loxP and n =2 IR loxP/loxP ;Foxo1 loxP/loxP , L-Insulin Receptor KO includes n =6 and L-IRFoxo1DKO includes n =13, for fasting group. LWT group includes total of three mice with n =2 IR loxP/loxP and n =1 IR loxP/loxP ;Foxo1 loxP/loxP , L-Insulin Receptor KO includes n =3 and L-IRFoxo1DKO includes n =8 for 15 min group. **** P <0.0001 versus LWT, # to P <0.0001 vs L-Insulin Receptor KO ( h ) Intraperitoneal glucose tolerance test (2 g kg −1 ) on overnight fasted mice. n =7–10 mice. LWT group includes total of six mice with n =5 IR loxP/loxP and n =1 IR loxP/loxP ;Foxo1 loxP/loxP . L-Insulin Receptor KO includes n =8 and L-IRFoxo1DKO includes n =5. ** P <0.01 versus LWT, **** P <0.0001 versus LWT. All data are presented as mean±s.e.m. Statistical analysis was performed using one-way analysis of variance followed by Tukey post-test when more than two groups were compared, two-way analysis of variance followed by Bonferroni when two conditions were involved. A P <0.05 was considered statistically significant. Full size image Insulin suppresses HGP in vivo in L-IRFoxo1DKO mice Despite the lack of hepatic insulin signalling in L-IRFoxo1DKO, the wild-type fasting glucose and insulin levels suggest these mice have normal HGP. However, these data do not provide information about the ability of insulin to regulate HGP. To ascertain whole-body insulin sensitivity directly and determine if insulin can suppress HGP independent of liver insulin signalling, hyperinsulinemic-euglycemic clamps in awake, unrestrained mice were performed. During insulin infusion under glucose clamp conditions, L-Insulin Receptor KO mice displayed a lower glucose infusion rate ( Fig. 3a ), a 25% decrease in glucose disposal ( Fig. 3b ) and a failure to suppress hepatic glucose production ( Fig. 3c,d ) compared with LWT mice. Concomitant deletion of Foxo1 in L-IRFoxo1DKO mice normalized the glucose infusion rate ( Fig. 3a ) confirming that Foxo1 deletion reversed the insulin resistance conferred by loss of the IR . L-IRFoxo1DKO mice had a normal rate of glucose disposal ( Fig. 3b ) and, most importantly, insulin suppressed hepatic glucose production to the same extent as in LWT mice ( Fig. 3c,d ). As noted previously, in this hyperinsulinemic–euglycemic clamp paradigm, insulin reduced glucose-6-phosphatase ( G6pc) without affecting phosphoenolpyruvate carboxykinase ( Pck1 ) expression in wild-type mice ( Fig. 3f ) [6] . At the end of the clamp procedure, levels of G6pc and Pck1 in L-Insulin Receptor KO mice were significantly elevated compared with both LWT and L-IRFoxo1DKO mice ( Fig. 3g ). The data support the hypothesis that insulin signals via an extrahepatic tissue to regulate hepatic glucose production and the expression of G6pc . 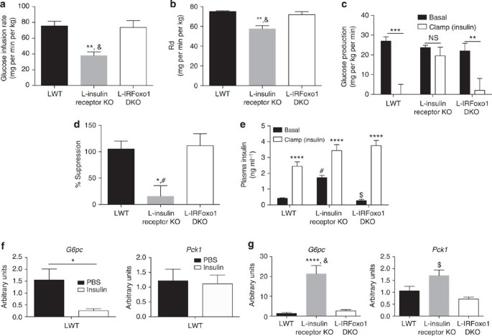Figure 3: L-IRFoxo1DKO are insulin responsive during euglycemic clamps. Hyperinsulinemic-euglycemic clamps were perfromed on unrestrained 5 h fasted mice using a 2.5 mU ming−1kg−1infusion of insulin. (a) Steady state glucose infusion rate (b) rate of glucose disposal (c) hepatic glucose production during basal and insulin portions of the clamp (d) percent suppression of hepatic glucose production during the clamp portion compared to basal period (e) insulin levels during during basal and insulin portions of the clamp. *P<0.05 versus LWT, **P<0.01 versus LWT, ***P<0.001 versus LWT, ****P<0.0001 versus LWT #P<0.05 versus Insulin Receptor KO, &P<0.01 versus L-Insulin Receptor KO, $P<0.0001 versus L-Insulin Receptor KO. LWT group includes total of 4 mice withn=2IRloxP/loxPandn=2IRloxP/loxP;Foxo1loxP/loxP. L-Insulin Receptor KO includesn=6 and L-IRFoxo1DKO includesn=4. ****P<0.0001 versus LWT $P<0.0001 versus L-Insulin Receptor KO. (f) Relative expression ofG6pcandPck1under euglycemic conditions with/without infusion of 2.5 mU ming−1kg−1of insulin for 120 min. *P<0.05 versus PBS of indicated genotype.n=3 (PBS),n=6 (insulin). (g) Relative expression ofG6pcandPck1under euglycemic conditions with infusion of 2.5 mU ming−1kg−1of insulin for 120 min. LWT group includes total of 4 mice withn=2IRloxP/loxPandn=2IRloxP/loxP;Foxo1loxP/loxP. L-Insulin Receptor KO includesn=4 and L-IRFoxo1DKO includesn=4. ****P<0.0001 versus LWT $P<0.0001 versus L-Insulin Receptor KO. All data are presented as mean±s.e.m. Statistical analysis was performed using one-way analysis of variance followed by Tukey post-test. AP<0.05 was considered statistically significant. Figure 3: L-IRFoxo1DKO are insulin responsive during euglycemic clamps. Hyperinsulinemic-euglycemic clamps were perfromed on unrestrained 5 h fasted mice using a 2.5 mU ming −1 kg −1 infusion of insulin. ( a ) Steady state glucose infusion rate ( b ) rate of glucose disposal ( c ) hepatic glucose production during basal and insulin portions of the clamp ( d ) percent suppression of hepatic glucose production during the clamp portion compared to basal period ( e ) insulin levels during during basal and insulin portions of the clamp. * P <0.05 versus LWT, ** P <0.01 versus LWT, *** P <0.001 versus LWT, **** P <0.0001 versus LWT # P <0.05 versus Insulin Receptor KO, & P <0.01 versus L-Insulin Receptor KO, $ P <0.0001 versus L-Insulin Receptor KO. LWT group includes total of 4 mice with n =2 IR loxP/loxP and n =2 IR loxP/loxP ;Foxo1 loxP/loxP . L-Insulin Receptor KO includes n =6 and L-IRFoxo1DKO includes n =4. **** P <0.0001 versus LWT $ P <0.0001 versus L-Insulin Receptor KO. ( f ) Relative expression of G6pc and Pck1 under euglycemic conditions with/without infusion of 2.5 mU ming −1 kg −1 of insulin for 120 min. * P <0.05 versus PBS of indicated genotype. n =3 (PBS), n =6 (insulin). ( g ) Relative expression of G6pc and Pck1 under euglycemic conditions with infusion of 2.5 mU ming −1 kg −1 of insulin for 120 min. LWT group includes total of 4 mice with n =2 IR loxP/loxP and n =2 IR loxP/loxP ;Foxo1 loxP/loxP . L-Insulin Receptor KO includes n =4 and L-IRFoxo1DKO includes n =4. **** P <0.0001 versus LWT $ P <0.0001 versus L-Insulin Receptor KO. All data are presented as mean±s.e.m. Statistical analysis was performed using one-way analysis of variance followed by Tukey post-test. A P <0.05 was considered statistically significant. Full size image Feeding suppresses gluconeogenic genes in L-IRFoxo1DKO mice L-IRFoxo1DKO mice are glucose tolerant and insulin suppresses hepatic glucose production despite lacking hepatic insulin signalling. These data support previous observations that mice lacking Akt isoforms and Foxo1 in the liver can respond to insulin to reduce glucose production and transition to the fed state [17] . In addition to rescuing the defects in glucose metabolism, deletion of Foxo1 restored the inability of both the Irs and Akt liver double knockouts to regulate genes involved in gluconeogenesis [15] , [17] . To test if hepatic insulin action is required for the changes in gene expression in response to feeding, mice were subjected to an overnight fast and refed. In LWT mice, 4 h after refeeding there was the expected gene changes in expression, with suppression of G6pc , Pck1 , Igfbp1 and induction of Srebp1c and Gck ( Fig. 4 ). Similar to previous models of defective hepatic insulin action, L-Insulin Receptor KO mice failed to reduce G6pc , Pck1 or increase Srebp1 and Gck mRNA in response to feeding; in addition, there was augmented expression of the Foxo1 target genes Igfbp1 and Irs2 ( Fig. 4 ). Despite the loss of hepatic insulin signalling in L-IRFoxo1DKO mice, refeeding suppressed both G6pc and Pck1 expression but failed to induce Srebp1 and Gck expression ( Fig. 4 ). Thus, hepatic insulin signalling is dispensable for the normal prandial response on gluconeogenic genes yet is required for the induction of Gck and the master lipogenic transcription factor, Srebp1c . 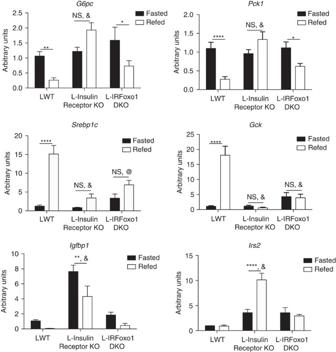Figure 4: Metabolic transcriptional response to feeding in the absense of hepatic insulin signaling. Hepatic gene expression in LWT, L-Insulin Receptor KO, and L-IRFoxo1DKO following an overnight fast and 4 h of refeeding normal chow. LWT group includes total of 9 mice withn=5IRloxP/loxPandn=4IRloxP/loxP;Foxo1loxP/loxP. L-Insulin Receptor KO includesn=6 and L-IRFoxo1DKO includesn=4-5 *P<0.05 versus fasted condition of indicated genotype, **P<0.01 versus fasted condition of indicated genotype, ****P<0.0001 versus fasted condition of indicated genotype, #P<0.0001 versus fasted LWT, @P<0.001 versus fed LWT. All data are presented as mean±s.e.m. Statistical analysis was performed using two-way analysis of variance followed by Bonferroni post-test. AP<0.05 was considered statistically significant. Figure 4: Metabolic transcriptional response to feeding in the absense of hepatic insulin signaling. Hepatic gene expression in LWT, L-Insulin Receptor KO, and L-IRFoxo1DKO following an overnight fast and 4 h of refeeding normal chow. LWT group includes total of 9 mice with n =5 IR loxP/loxP and n =4 IR loxP/loxP ;Foxo1 loxP/loxP . L-Insulin Receptor KO includes n =6 and L-IRFoxo1DKO includes n =4-5 * P <0.05 versus fasted condition of indicated genotype, ** P <0.01 versus fasted condition of indicated genotype, **** P <0.0001 versus fasted condition of indicated genotype, # P <0.0001 versus fasted LWT, @ P <0.001 versus fed LWT. All data are presented as mean±s.e.m. Statistical analysis was performed using two-way analysis of variance followed by Bonferroni post-test. A P <0.05 was considered statistically significant. Full size image Insulin fails to suppress genes in vitro in L-IRFoxo1DKO mice To confirm that insulin was acting cell-non-autonomously to regulate HGP and gluconeogenic genes in L-IRFoxo1DKO mice, primary hepatocytes were isolated from LWT, L-Insulin Receptor KO and L-IRFoxo1DKO mice. Glucose production was measured over 6 h in response to db-cAMP, insulin and db-cAMP and insulin. In all genotypes, db-cAMP stimulated glucose production approximately 30–40% ( Fig. 5a ). L-Insulin Receptor KO mice exhibited increased glucose production that was normalized with concomitant Foxo1 deletion during all treatments ( Fig. 5a ). G6pc and Pck1 expression was induced in response to db-cAMP in both LWT and L-Insulin Receptor KO. However, L-IRFoxo1DKO mice exhibited a defect in gluconeogenic gene expression in response to db-cAMP ( Fig. 5b ). Insulin did not affect glucose production in isolated hepatocytes in any genotype or condition. However, insulin significantly reduced G6pc , Pck1 and Igfbp1 mRNA in hepatocytes isolated from LWT but not from L-Insulin Receptor KO or L-IRFoxo1DKO mice. 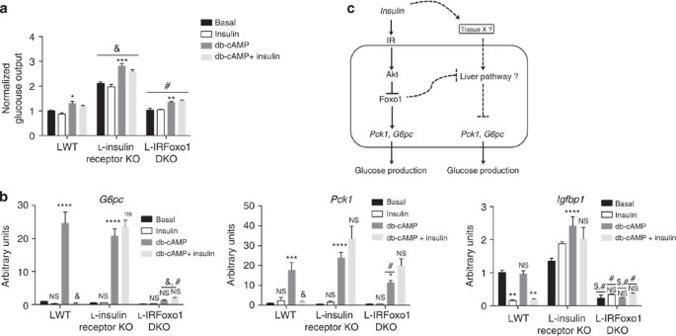Figure 5: Glucose production and gluconeogenic gene response to insulin and cAMP in isolated primary hepatocytes. Primary hepatocytes were isolated from indicated genotype and treated with either 0.1 mM db-cAMP and/or 0.1 μM insulin for 6 h. (a) Glucose concentration in media was determined and expressed normalized to protein concentration. (b) Gene expression analysis was performed at the end of the treatments. Data is from a representative experiment and presented as mean±s.e.m.. *P<0.05 versus basal condition of indicated genotype, **P<0.01 versus basal condition of indicated genotype, ***P<0.001 versus basal condition of indicated genotype, ****P<0.001 versus basal condition of indicated genotype , #P<0.0001 versus L-Insulin Receptor KO, &P<0.0001 versus LWT for indicated treatment condition. All data are presented as mean±s.e.m. Statistical analysis was performed using two-way analysis of variance followed by Bonferroni post-test. AP<0.05 was considered statistically significant. (c) In hepatocytes, insulin stimulates the kinase Akt thus inactivating the transcription factor Foxo1, which leads to the suppression of gluconeogenic genes and glucose production. In addition to the canonical IR-Akt liver pathway, there is an insulin responsive non-hepatic tissue (tissue X) capable of communicating with the liver to regulate hepatic glucose output and gluconeogenic genes. An unidentified liver pathway receives the insulin signal via tissue X to suppress gluconeogenic genes and glucose output in response to insulin. Deletion in liver of theIR, Irs, orAktgene or high fat diet feeding leads to abberant Foxo1 activity, which represses this unidentified liver pathway. Ablation of hepaticFoxo1alleviates this suppressive effect allowing insulin to regulate hepatic glucose metabolism. Figure 5: Glucose production and gluconeogenic gene response to insulin and cAMP in isolated primary hepatocytes. Primary hepatocytes were isolated from indicated genotype and treated with either 0.1 mM db-cAMP and/or 0.1 μM insulin for 6 h. ( a ) Glucose concentration in media was determined and expressed normalized to protein concentration. ( b ) Gene expression analysis was performed at the end of the treatments. Data is from a representative experiment and presented as mean±s.e.m.. * P <0.05 versus basal condition of indicated genotype, ** P <0.01 versus basal condition of indicated genotype, *** P <0.001 versus basal condition of indicated genotype, **** P <0.001 versus basal condition of indicated genotype , # P <0.0001 versus L-Insulin Receptor KO, & P <0.0001 versus LWT for indicated treatment condition. All data are presented as mean±s.e.m. Statistical analysis was performed using two-way analysis of variance followed by Bonferroni post-test. A P <0.05 was considered statistically significant. ( c ) In hepatocytes, insulin stimulates the kinase Akt thus inactivating the transcription factor Foxo1, which leads to the suppression of gluconeogenic genes and glucose production. In addition to the canonical IR-Akt liver pathway, there is an insulin responsive non-hepatic tissue (tissue X) capable of communicating with the liver to regulate hepatic glucose output and gluconeogenic genes. An unidentified liver pathway receives the insulin signal via tissue X to suppress gluconeogenic genes and glucose output in response to insulin. Deletion in liver of the IR, Irs , or Akt gene or high fat diet feeding leads to abberant Foxo1 activity, which represses this unidentified liver pathway. Ablation of hepatic Foxo1 alleviates this suppressive effect allowing insulin to regulate hepatic glucose metabolism. Full size image In this study, we used genetic loss of function experiments in mice to test the requirement for hepatic insulin action for the insulin-dependent regulation of glucose metabolism and transcription in mouse liver. Data presented herein confirm previous studies that signalling via the hepatic insulin receptor is essential for normal glucose metabolism in adult mice [18] . Substantial data support a model in which insulin regulates glucose metabolism by signalling through Akt-mediated inactivation of the transcription factor, Foxo1, thus contributing to the metabolic transition that accompanies the intake of food. Nonetheless, insulin suppressed hepatic glucose output during euglycemic clamps in mice with livers deficient for the IR and Foxo1. These data refute the idea that the canonical model of hepatic insulin action in liver represents the exclusive pathway by which the hormone suppresses hepatic glucose output. Moreover, the persistence of hepatic effects of insulin in L-IRFoxo1DKO mice strongly supports the hypothesis that, at least under some conditions, insulin can act cell non-autonomously to suppress hepatic glucose output and regulate gene expression [17] . The hypothesis that indirect mechanisms contribute to the regulation of insulin mediated suppression of HGP dates back almost 60 years [21] . In support of this idea, restoring hepatic insulin signalling is not sufficient to fully suppress HGP in mice with systemic loss of the insulin receptor [22] . Data presented herein provide genetic evidence that insulin uses both an intra- and extrahepatic mechanisms to regulate liver metabolism. Previous studies using liver-specific insulin receptor knockout (LIRKO) mice have reported robust defects in glucose homeostasis and peripheral insulin resistance [18] , [23] . LIRKO mice develop profound insulin resistance as adults; however, the lack of the insulin receptor from birth also leads to liver failure in aged mice. To avoid the complications of congenital liver-specific deletion, we employed a model that relies on acute deletion of the insulin receptor in adult mice [8] . L-Insulin Receptor KO mice displayed mild glucose intolerance and insulin resistance without the confounding peripheral insulin resistance and pronounced fasting hyperglycaemia in the LIRKO mice. Moreover, the mild hyperglycaemia of the acute IR deletion was less severe than in acute liver-specific deletion of both Akt isoforms [17] . This difference in severity may be due to significant basal Akt activity independent of insulin action, leading to partial inhibition of Foxo1, even in fasting, non-obese mice [17] . Considerable data refute the idea that insulin signals though a hepatocyte, cell autonomous pathway in L-IRFoxo1DKO mice. Insulin failed to promote phosphorylation of the canonical targets Akt and S6 in L-Insulin Receptor KO and L-IRFoxo1DKO mice. Though it has been suggested that IGF1-R can be induced in liver by stresses such as regeneration [24] , we did not detect IGF1-R protein in livers from LWT, L-Insulin Receptor KO or L-IRFoxo1DKO mice ( Fig. 2a ). High concentrations of insulin were completely without effect on isolated hepatocytes lacking insulin receptors with or without concomitant deletion of Foxo1 ( Fig. 5b ). One of the major unanswered questions that arise from this study is the identity of the extrahepatic tissue that is binding insulin and transmitting the signal to suppress hepatic glucose output and gluconeogenic gene expression. On the basis of recent work, perhaps the most likely site of insulin action is the central nervous system (CNS), which has been proposed to serve as an organizing centre for metabolic control [25] , [26] , [27] . In support of a direct communication between the CNS and liver, intracerebral ventricular infusion of insulin suppresses HGP without activation of hepatic insulin signalling through the hepatic vagus nerve [28] , [29] . Moreover, mice with insulin receptor deficiency in AgRP neurons fail to suppress HGP in response to peripheral insulin infusion during euglycemic clamps [30] . However, infusion of insulin in the brain of dogs only increases liver glycogen synthesis without affecting glucose output, questioning the significance of a CNS mechanisms in the regulation of HGP [31] , [32] . Future studies are needed to assess the contribution of insulin action in the CNS to the regulation of HGP in mice with livers lacking autonomous insulin action. In addition to the CNS, a more classical target of insulin action is adipose tissue. It has been hypothesized that the insulin-dependent suppression of lipolysis limits gluconeogenesis by reduction in circulating glycerol and free fatty acids [33] . Preventing the fall of free fatty acids during hyperinsulinemic–euglycemic clamps by infusing a lipid/heparin mixture antagonizes the reduction of hepatic glucose output in dogs [34] . Moreover, pharmacological suppression of lipolysis alone is sufficient to reduce HGP independent of changes in insulin levels [35] . The other well-established pathway for regulating HGP is through the counter-regulatory hormone glucagon, whose secretion by the alpha cells of the pancreas is itself reduced by insulin [3] , [36] . Indeed, the decline in portal glucagon concentrations during hyperinsulinemic–euglycemic clamps in dogs correlates well with reductions in HGP [37] . However, a reduction in peripheral glucagon during clamp experiments in mice has been difficult to observe [23] . Defining the relative contributions of these cell non-autonomous pathways for the regulation of HGP by insulin will be of significant interest. Since these data establish an extrahepatic pathway in the regulation of HGP, there must exist a liver autonomous mechanism to receive the signal initiated by insulin’s interaction with a non-hepatic tissue. In L-Insulin Receptor KO mice, this unidentified liver autonomous pathway is suppressed by aberrant Foxo1 activity, preventing insulin’s regulation of hepatic glucose output. On deletion of Foxo1 , as in L-IRFoxo1DKO mice, the suppressive effect of Foxo1 on this pathway is lost allowing insulin to signal to the liver via an intermediary peripheral tissue to suppress hepatic glucose output and gluconeogenic gene expression ( Fig. 5c ). The identity of this pathway remains unknown and presents a novel therapeutic target for the regulation of HGP independent of hepatic insulin action. Though deletion of Foxo1 in IR null livers restored the response of gluconeogenic genes to nutritional regulation, lipogenic genes such as Srebp1c and Gck remained unresponsive to refeeding in the absence of hepatic insulin receptors ( Fig. 4 ). Following a meal, insulin and nutrients activate the mTORC1 signalling pathway that leads to increased lipogenesis and lipogenic gene expression, in part by inducing the transcription and posttranslational processing of SREBP1c [8] , [38] . However, refeeding fails to increase Srebp1c and Gck gene expression in the liver of L-IRFoxo1DKO to the same extent as LWT mice. Indeed, the hepatic insulin receptor is required for SREBP1c induction and de novo lipogenesis in vivo [20] . The failure to induce lipogenic genes in L-IRFoxo1DKO mice suggests strongly that insulin can stimulate lipid synthesis only by a cell autonomous pathway. In summary, we have demonstrated that the abnormal hepatic glucose metabolism and insulin resistance resulting from lack of hepatic insulin receptor is dependent on a constitutively active Foxo1. On Foxo1 deletion, the insulin-dependent regulation of glucose metabolism in vivo was largely restored, supporting the idea that reducing Foxo1 activity in insulin resistant disorders may have beneficial effects [16] , [39] . In addition, we provided genetic evidence that an extra-hepatic insulin-responsive tissue communicates with the liver to regulate glucose output. Elucidation of this pathway may provide a novel target for the treatment of insulin resistant disorders such as diabetes mellitus. Mice Male mice were used in all experiments. The IR loxP/loxP and Foxo1 loxP/loxP mice were described previously [11] , [40] . IR loxP/loxP ;Foxo1 loxP/loxP mice were generated by crossing the IR loxP/loxP (C57Bl/6J) with the Foxo1 loxP/loxP (FVB) mice. These mice were on a 129-C57BL/6J-FVB mixed background. Mice were injected at 6- to 8-weeks of age with 10 11 genomic copies per mouse with adeno-associated-virus containing a liver-specific promoter, thyroxine-binding globulin (TBG) promoter driving either GFP or Cre recombinase to generate LWT, L-Insulin Receptor KO, or L-IRFoxo1DKO [8] . The LWT group consisted of pooled GFP injected IR loxP/loxP and IR loxP/loxP ;Foxo1 loxP/loxP mice. GFP injected IR loxP/loxP and IR loxP/loxP ;Foxo1 loxP/loxP mice did not significantly differ in any observed measurement therefore data is shown as the pooled averages from both genotypes. Experiments were performed 2–3 weeks after virus injection. To generate liver-specific congenital knockouts, IR loxP/loxP and IR loxP/loxP ;Foxo1 loxP/loxP mice were crossed to an Alb-Afp-cre mouse [41] (kind gift from Klaus Kaestner) and littermate floxed mice served as controls. For the fasting and refeeding experiments, mice were deprived of food for 16 h overnight, then killed (for the fasted groups) or refed with normal chow (Laboratory Rodent Diet 5,001) for an additional 4 h before killing (for the refed group). For insulin injection, 16-h fasted mice were i.p. injected with 3% bovine serum albumin in saline or insulin at 2 mU g −1 of body weight 20 min before killing the mice and excising the liver for rapid freezing in liquid nitrogen. All mice experiments were reviewed and approved by the University of Pennsylvania Institutional Animal Care and Use Committee in accordance with the guidelines of the National Institutes of Health. Liver protein extraction and western blotting Livers were freeze clamped and stored at −80 °C until further processing. Protein lysates were extracted from frozen livers with a modified RIPA buffer (150 mM NaCl, 50 mM Tris, pH 7.6, 1% Triton X-100, 0.5% sodium deoxycholate and 0.1% SDS, supplemented with protease (Roche) and phosphatase (Sigma) inhibitors. Cleared supernatants were extracted from cellular debris following 15-min centrifugation at 17,000 g . The following antibodies were used for immunoblotting at a dilution of 1:1,000: insulin receptor, IGF1-R, Foxo1, p-Ser 473 Akt, Akt, pPRAS 40, PRAS, p-S6 Ser 240 and Ser 244, S6 were from Cell Signaling Technology; antibody to Igfbp1 was purchased from Santa Cruz Biotechnology; antibodies to GFP and tubulin were from Sigma; antibody to Gck was provided by M.A. Magnuson (Vanderbilt University). Complete scans of key immunoblots are provided in Supplementary Fig. 1 . mRNA isolation and real-time PCR Total RNA was isolated from frozen livers using the NucleoSpin RNA kit from Clontech. Complementary DNA was synthesized using Moloney murine leukaemia virus reverse transcriptase and the relative expression of the genes of interest was quantified by real-time PCR using the SYBR Green Dye-based assay. Primer sequences are provided in Supplementary Table 1 . Primary hepatocytes isolation Hepatocytes were isolated from random fed mice using a two-step collagenase/DNAse digestion protocol [42] . For glucose output studies, primary hepatocytes from indicated genotypes were isolated and plated in M199 media containing 10% FBS, 100 nM T3, 500 nM dexamethasone and 1 nM insulin. Following attachment, cells were changed to M199 media containing 100 nM dexamethasone, and 1 nM insulin were indicated and incubated overnight. Cells were washed switched to glucose output media (DMEM no glucose) and incubated with 10 mM lactate 1 mM pyruvate, 100 nM dexamethasone and 100 nM insulin and/or 100 uM db-cAMP were indicated. Glucose production was determined by the measurement of glucose in the media over a 6 h time course using hexokinase glucose assay. Cells were lysed in modified RIPA buffer described above and subjected to western blot analysis or protein normalization for glucose output studies. Alternatively, cells were harvested for RNA isolation and subsequent gene expression analysis as described above. Metabolic measurements For glucose tolerance test, overnight fasted mice were given glucose at 2 g kg −1 body weight via intraperitoneal injection. Blood glucose concentrations in the mice were monitored by tail bleeding at 0, 15, 30, 60 and 120 min after glucose injection. Insulin concentrations were measured from plasma collected from the mice before and 15 min following glucose injection. Hyperinsulinemic-euglycemic clamp Euglycemic clamps were performed on unrestrained and awake 8–10-week-old mice [6] . Indwelling catheters were placed into mice 5–7 days prior to clamp experiments. Mice were fasted for 4 h and a priming 5 μCi [3-3H]glucose (Perkin Elmer HPLC purified) bolus followed by 0.05 μCi/min infusion was initiated for 120 min. Following the basal period, mice were given a bolus of 150 mU kg −1 insulin (or PBS) and a 0.1 μCi min −1 [3-3H]glucose infusion with insulin was initiated (6 h from start of fast). The rate of insulin infusion was 2.5 mU kg −1 min −1 , and the glucose infusion rate was adjusted to keep euglycemic levels between 100 and 130 mg dl −1 . PBS without glucose was infused in the control groups for gene expression analysis. Blood was taken by tail bleeding, and blood glucose levels were measured every 10 min during the clamp. Rd and HGP were calculated from the blood sampling every 10 min during the steady state portion of (80–120 min). At the end of the 2-h clamp, mice were killed by pentobarbital injection, and livers were quickly removed, freeze clamped in liquid nitrogen and stored at −80 °C for future uses. Statistical analysis All data are presented as mean±s.e.m. Statistical analysis was performed using one-way analysis of variance followed by Tukey post-test when more than two groups were compared, two-way analysis of variance followed by Bonferroni post-test when two conditions were involved and a Students’s t test with two-tailed analysis when only two groups of data were concerned. A P <0.05 was considered statistically significant. How to cite this article: Titchenell, P. M. et al . Hepatic insulin signalling is dispensable for suppression of glucose output by insulin in vivo . Nat. Commun . 6:7078 doi: 10.1038/ncomms8078 (2015).